A few basic concepts in electrochemical carbon dioxide reduction In heterogeneous catalysis, periodic density functional theory (DFT) simulations have really enabled us to computationally explore reaction mechanisms. For electrocatalysis, the “computational hydrogen electrode” model is our standard method to determine reaction thermodynamics [9] . This method trivially translates simulations in vacuum to potential-dependent energetics, without requiring we simulate explicitly the ions or potential. Our models of the electrolyte and electrochemical reaction barriers, in contrast, are far from convergent. Our field abounds with different approaches towards the electrolyte: implicit continuum models, explicit ab initio ones, or a hybrid of the two (Fig. 1a ) [10] . We also have multiple ways to obtain the potential and the potential dependence of the reaction energetics [11] . While continuum approximations give us huge reductions in computational cost, we see significant deviations in solvation energies determined with implicit vs. dynamic explicit water models [12] . Furthermore, different ways to set up the applied potential result in differences in the computed reaction energetics [13] . All these challenges could contribute to the wide range in the computed energetics and mechanisms towards the various C 2 products [1] . Fig. 1: Some basic ideas from mechanistic studies of electrochemical carbon dioxide reduction. a Implicit, explicit, and hybrid approaches to model the electrolyte in ab initio simulations. b In electrochemical reactions with multiple proton–electron transfers, the number of electrons n transferred prior to the rate-limiting step determines both the Tafel slope and how changes in pH shift the activity. c Rate-limiting steps for CO 2 reduction to CO (on weak binding catalysts) and C 2 products (on Cu) involve intermediates with large dipole moments μ , which interact with the interfacial electric field E . d The absolute potential (e.g., U vs. SHE) determines the electric field at an electrochemical interface and the corresponding stabilization of the polar *CO 2 and *OCCO intermediates. Since the dipoles point away from the interface, the field-stabilization occurs at potentials below the potential of zero charge. A given field stabilization corresponds to a more positive overpotential at higher pH (e.g., a 360 mV shift between pH 7 and 13), which leads to higher CO (2) R activity at higher pH. e The differences in hydrated cation sizes (e.g. hydrated Li + vs. hydrated Cs + ) lead to differences in the surface charge density and interfacial field at a given applied potential. This model is an example of the Frumkin effect: the interfacial field (or equivalently the local potential drop) is the driving force for electrochemical processes, and different compositions of the electric double layer give rise to different fields at a given applied potential. Full size image Despite the difficulties in an ab initio treatment of electrochemical reaction barriers, we do need kinetics for mechanistic understanding. Case in point: our evolving understanding of CO (2) R to CH 4 on Cu [14] . A thermodynamic analysis showed a proton–electron transfer to *CO to form *CHO to be the rate-limiting step. Considering the corresponding barriers across different materials, we suggested the transition state of this process to be the descriptor of activity. But when we simply consider the kinetics of electrochemical reactions with multiple proton–electron transfers, we see that this step cannot be rate limiting on Cu . 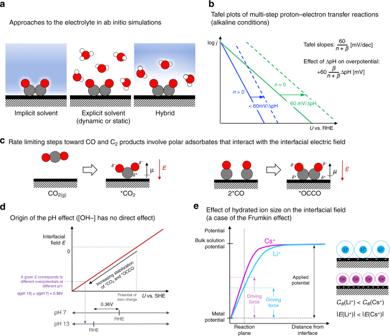Fig. 1: Some basic ideas from mechanistic studies of electrochemical carbon dioxide reduction. aImplicit, explicit, and hybrid approaches to model the electrolyte in ab initio simulations.bIn electrochemical reactions with multiple proton–electron transfers, the number of electronsntransferred prior to the rate-limiting step determines both the Tafel slope and how changes in pH shift the activity.cRate-limiting steps for CO2reduction to CO (on weak binding catalysts) and C2products (on Cu) involve intermediates with large dipole momentsμ, which interact with the interfacial electric fieldE.dThe absolute potential (e.g.,Uvs. SHE) determines the electric field at an electrochemical interface and the corresponding stabilization of the polar *CO2and *OCCO intermediates. Since the dipoles point away from the interface, the field-stabilization occurs at potentials below the potential of zero charge. A given field stabilization corresponds to a morepositiveoverpotential at higher pH (e.g., a 360 mV shift between pH 7 and 13), which leads to higher CO(2)R activity at higher pH.eThe differences in hydrated cation sizes (e.g. hydrated Li+vs. hydrated Cs+) lead to differences in the surface charge density and interfacial field at a given applied potential. This model is an example of the Frumkin effect: the interfacial field (or equivalently the local potential drop) is the driving force for electrochemical processes, and different compositions of the electric double layer give rise to different fields at a given applied potential. The corresponding Tafel plots have defining features that depend on the symmetry factor β (0 < β < 1) for the rate-limiting step, as well as the number of proton–electron transfers preceding it, n. Figure 1b shows the Tafel slopes and the effect of pH on the overpotential for alkaline solutions, where H 2 O as the proton donor. Experiments show CH 4 activity to have a Tafel slope of <60 mV/dec, and the positive shift in overpotential with an increased pH is <60 mV/pH unit, both consistent with n > 0. Therefore, the rate-limiting step must occur after the initial proton–electron transfer to *CO to form *CHO (or *COH [15] ) . And Hori, in fact, made these observations decades ago [8] . To put some numbers on what we can do today, consider the Arrhenius law, 
    TOF = Aexp(  - E_a/kT),
 (1) where A is the prefactor, TOF the turnover frequency, and E a the activation energy. Without even considering the electrochemical environment, a typical DFT error in adsorption energy is 0.15 eV [16] . A shift in E a of this magnitude gives a 300× change in the TOF at room temperature! Depending on the reaction process at play, the corresponding theoretical selectivities can have uncertainties that approach 100% [17] . With electrochemical barriers, the uncertainties are compounded by the challenges mentioned above. So DFT-based kinetic models do not presently give us predictions of activity or selectivity to the precision of experiments where mass transport and the surface structure of the catalyst are carefully controlled. With error cancellation, we have much more confidence in the relative : the relative magnitudes of barriers within a given mechanism, as well as the relative activity across catalysts [16] and across reaction conditions [18] . Especially with our present degree of accuracy, we should, wherever possible, couple DFT models to ample feedback from experiment. Such joint efforts have given us valuable insights into reaction mechanisms, activity descriptors, and electrolyte effects [1] . The activity towards CO and C 2 products is driven by field–dipole interactions A special feature of CO (2) R is the importance of steps that do not involve a proton–electron transfer (Fig. 1c ). On weak binding catalysts (e.g. Au [19] and Fe-N-C [20] catalysts), the rate of CO 2 R to CO is limited by CO 2 adsorption. On Cu catalysts, CO–CO coupling limits the rate of CO (2) reduction to high-value C 2 products such as ethanol and ethylene [3] . Now, the dipoles of *CO 2 and *OCCO interact strongly with the interfacial electric field. And since the field depends on the absolute potential, e.g. on an SHE scale, so does the activity of the corresponding reactions. Figure 1d shows the variation of the interfacial field E and the corresponding stabilization of the polar intermediates vs. the potential U vs. SHE. On the other hand, the overpotential η depends on U vs. RHE, which shifts on the SHE scale by a Nernstian factor of 60 mV/pH unit. For reduction reactions, a positive shift in η translates to higher activity. For example, a shift in pH from 7 to 13 translates to a whopping shift in η of +0.36 V! We can therefore think of the dramatic pH effect for these products as simply arising from a shift in the RHE reference potential. We can use different labels for this phenomenon, such as single electron transfer [19] or decoupled proton–electron transfer [3] , but the dipole-field vocabulary allows us to consider the reaction rate in terms of dipoles of the intermediates, μ , and the interfacial capacitance, C dl . For example, the rate of CO 2 adsorption and the corresponding Tafel slope are as follows [21] , [22] : 
    j ∝exp(  - μ( CO_2)_TS· E/kT),
 (2) 
    Tafel slope = | ∂ U/∂log j| ∝1/μ( CO_2)_TSC_dl
 (3) and we can write analogous expressions for CO dimerization. Note that the local [OH – ], which increases with increasing CO (2) R current, plays no direct role in promoting the rate of these two steps [23] , since they are driven by the field alone . However, the [OH – ] can alter the CO 2 concentration through the bicarbonate equilibria, suppress CH 4 formation [14] , and promote the activity towards acetate, even at a fixed U vs. SHE [24] . These very dipole–field interactions also rationalize the sensitivity of activity to cation identity [18] (Fig. 1e ). In a classical picture of the interface, the ion concentration is limited by the hydrated ion size [25] . The smaller the size, the greater the surface charge and interfacial field for a given applied potential, which increases C dl . The slightly smaller hydrated size of Cs + vs. Li + leads to the 1–2 orders of magnitude enhancement for the CO activity on Ag and C 2 activity on Cu. This model of the ion effects is an echo of the decades-old “Frumkin diffuse layer correction” to Butler–Volmer kinetics [26] . This correction accounts for the impact of the composition of the double layer on the local potential drop, which determines the corresponding reaction rate. Beyond electrostatics, specific chemical interactions between ions with the surface or adsorbate may also play a role, and both cations and anions can act as buffers [27] , [28] . The dependence of CO (2) R on adsorbate–field interactions shows us that, in addition to optimizing the adsorption energies of critical intermediates, we can look to tuning C dl and μ towards higher activity (Eq. 3 ). Our models suggest that we can tune the former through the electrolyte, and the latter in single-atom catalysts, where the localization of charge on the active site is affected by the coordinating atoms [22] . What do we know about the activity of existing catalysts? Selectivities are often represented by Faradaic efficiencies: \({\mathrm{FE}}_{\mathrm{i}} = \frac{{j_i}}{{j_{{\mathrm{{tot}}}}}}\) , where j i is the partial current density of product i and j tot the total current density. While selectivities are a critical performance metric, FE i ’s can’t be used to evaluate the intrinsic activity towards a given product, especially as they shift with respect to changes in the activities of all other products. The intrinsic activity, as determined by the reaction energetics, can really only be evaluated by TOFs (Eq. 1 ). In practice, we approximate TOFs by partial current densities normalized to the electrochemically active surface area (ECSA), \(j_{{\mathrm{{ECSA}}}} \propto \rho _{{\mathrm{{site}}}}{\mathrm{TOF}}\) , where ρ site is the density of the active site. Comparisons of intrinsic activity with j ECSA are therefore accurate within the variations of ρ site among samples, the uncertainty in the ECSA, and the degree of mass transport limitations. Surface reaction energetics on different facets typically differ by 0.1–1 eV [29] , which translates to variations in the corresponding TOFs by orders of magnitude (Eq. 1 ). Shifts in j ECSA of around an order of magnitude (or less) between catalysts with different surface structures are more likely to arise from a change in ρ site than a change in the predominant active site or facet. Recent reviews have shown that nano-structured Cu and Cu-based bimetallics show similar j ECSA to those on Cu foils [1] , [2] . To date, I am not aware of a new catalyst with intrinsic activity towards C 2 products that unequivocally exceeds that of Cu foil. Ongoing efforts to obtain single crystal measurements with product quantification can rigorously evaluate theoretical predictions of the most active Cu facet(s). The increased C 2 selectivities on various high surface area Cu catalysts actually arise from the suppression of other products, such as CH 4 and H 2 [1] , [2] . Under alkaline conditions, H 2 suppression cannot arise from local changes in pH, since H 2 O is the proton donor. Perhaps nanostructuring shifts the structure and activity of water, such that products that are limited by proton–electron transfer steps are suppressed. And why haven’t we found alternatives to Cu that either match or exceed its intrinsic activity towards C 2 products? Stability is a possible culprit: leaching or surface restructuring, which can be driven by the presence of elements that strongly bind *CO. But I know no fundamental limitation on the existence of stable and active alternatives, especially if we expand our search to emergent classes of materials beyond binary combinations of transition metals [30] , [31] . Furthermore, improvements in catalytic efficiency are still needed [5] , [6] . With a rigorous consideration of surface stability, the discovery of new catalysts beyond Cu remains a worthwhile and important pursuit. Even as we develop practical devices and systems for CO 2 R, we still face fundamental challenges at the level of reaction mechanisms and intrinsic activity. These challenges range from simulating electrochemical kinetics to the discovery of new catalysts beyond Cu. Tremendous opportunity lies in overcoming them. With the increasing dialogue among us and the diversity of expertise we are bringing together—I envision that our collective efforts will ultimately contribute to establishing a sustainable carbon cycle.